Self-assembly of free-standing RNA membranes RNA has emerged as a promising material for nanostructure and microstructure engineering. Although rare, some macroscopic RNA structures have also been constructed using lipid or polymer materials. Here, we report the first example of an enzymatically generated RNA membrane. This robust and free-standing RNA membrane has a macroscopic structure and is generated without any polymer support or complexation. Our RNA membrane is fabricated following two sequential processes, complementary rolling circle transcription and evaporation-induced self-assembly, and its structural and functional properties are rationally controlled by adjusting RNA base pairing. In this study, three types of RNA membranes are fabricated and are used to demonstrate potential applications. Nucleic acids, deoxyribonucleic acid (DNA) and ribonucleic acid (RNA), have gained much attention as versatile materials for engineering nanoscale structures [1] , [2] , [3] , [4] , [5] . In the early 1990s, Seeman and colleagues first proposed using DNA to create self-assembling nanostructures [6] . Recently, DNA nanostructures have been used as novel functional biomaterials for various applications, such as multiplexed diagnosis [7] , [8] , [9] , gene and drug delivery [10] , [11] , [12] , [13] and molecular patterning [14] , [15] . In addition to its nanosized applications, DNA has been used for building micrometer-scale arrays [16] , [17] and even for centimeter-scale hydrogels as a mechanical metamaterial or for protein production [18] , [19] , [20] . Like DNA, RNA has been recently recognized as an effective material for constructing nanostructures with biological functions such as the catalytic activity characteristic of ribozymes [3] , [21] . RNA nanostructures have emerged as biologically functional nanomaterials for applications in nanomedicine, including the diagnosis and treatment of cancer, viral infection and genetic diseases [22] . Various RNA nanostructures, such as RNA nanorings [23] , branched RNAs [24] and packaging RNAs [25] , [26] have been developed to efficiently deliver RNA interference (RNAi) molecules, including small interfering RNA (siRNA), small hairpin RNA (shRNA) and microRNA (miRNA). RNA has also been shown to form micrometre-scale structures such as RNA-based microsponges [27] and siRNA microhydrogels [28] . Building on these previous achievements, the next challenge in RNA technology is to generate macroscopic RNA materials to explore the usage of RNA as a generic material. However, unlike DNA, there have been few reports on creating RNA membranes or hydrogels. There are only a few reports showing the preparation of RNA membranes via the ionic complexation of RNA with lipid or polymer [29] , [30] , in which the original properties of the RNA in the membrane can be reduced or eliminated by complexation with other materials. Therefore, a new approach to prepare RNA membranes without polymer supports or complexation is necessary. Our strategy was to generate membranes by enzymatic RNA polymerization. Here, we report the first example of a macroscopic RNA membrane composed of RNA strands. This RNA membrane is robust and self-standing ( Supplementary Fig. 1 ), and its structural and functional properties can be rationally controlled by adjusting the RNA base pairing. Based on the tunability of our membranes, controlled release of chemical molecules was observed. Because the sequences of RNA strands were easily changed, we could also engineer sequence-specific drug release systems. Especially, RNA membranes were designed to contain siRNA sequences to be cleaved by Dicer enzyme for siRNA release. Therefore, our RNA membrane may open a route in the development of RNA technology to create a novel biomaterial. RNA membrane fabrication To fabricate our RNA membrane, we chose a T7 RNA polymerase that is capable of RNA production. RNA polymerase uses a DNA strand as a template to generate single-stranded RNA transcripts [31] . Based on the enzymatic reaction of the RNA polymerase, we designed a combination of two sequential processes, a complementary rolling circle transcription (cRCT) reaction followed by an evaporation-induced self-assembly (EISA) [32] , [33] , [34] of RNA strands. After running the cRCT for 20 h followed by the EISA of the RNA strands, the efficient hybridization of two complementary RNA strands was performed to produce a RNA membrane ( Fig. 1 and Supplementary Fig. 2 ). Because the membrane was designed to be formed by the hybridization of RNA strands from the transcription of circular DNA, two complementary circular DNAs were first prepared ( Fig. 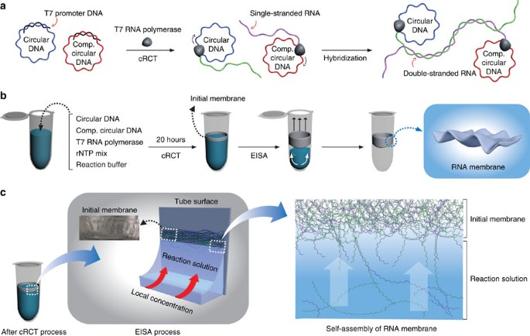Figure 1: Fabrication of a self-assembled free-standing RNA membrane. (a) Hybridization of RNA transcripts by the cRCT process. (b) Schematic drawing of the fabrication processes of the self-assembled RNA membrane. (c) Detailed description of the EISA by hybridization of the RNA strands of initial membrane and free RNA transcripts, resulting in self-assembly of the RNA membrane on the tube wall during the evaporation. Comp., complementary. 1a ; sequences in Supplementary Table 1 ). Following our previous publications [18] , [27] , the circular DNAs were synthesized with long linear DNA and the promoter DNA, which is required for the initiation of the rolling circle transcription (RCT) process ( Supplementary Fig. 3 ). Due to the partially complementary sequences of these two DNA strands, they were hybridized to form a circular shape. After hybridization, the nick was enzymatically closed by T4 DNA ligase [35] , [36] . Figure 1: Fabrication of a self-assembled free-standing RNA membrane. ( a ) Hybridization of RNA transcripts by the cRCT process. ( b ) Schematic drawing of the fabrication processes of the self-assembled RNA membrane. ( c ) Detailed description of the EISA by hybridization of the RNA strands of initial membrane and free RNA transcripts, resulting in self-assembly of the RNA membrane on the tube wall during the evaporation. Comp., complementary. Full size image With these two circular DNAs, we then assembled the RNA strands into large-area films by cRCT and EISA. Due to the complementary sequences of the RNA strands produced from cRCT, the rolling circle transcripts were hybridized to form a thin ring-like structure, named initial membrane, as an initiation process at the meniscus ( Fig. 1b,c ). As water evaporated after the cRCT process, the solution with RNA transcripts at the meniscus was thinned, forming concentrated water films in which the motions of the RNA strands were spatially confined to two dimensions by EISA ( Fig. 1c ). During this process, evaporation was greater near the air-solution-tube wall contact line [37] , resulting in local concentration and self-assembly of RNA strands on the tube wall at the meniscus. As a result, the RNA strands formed a large-area membrane on the inner wall ( Fig. 1b and Supplementary Fig. 2 ). Self-assembly of the RNA membranes The RNA membrane was fabricated by two sequential processes: cRCT and EISA. When the EISA process was finished, the macroscopic membrane was readily observed by the naked eye after staining with a GelRed ( Fig. 2a and Supplementary Movie 1 ). As expected, this stained membrane showed strong fluorescence, suggesting that the entire membrane was composed of RNA ( Fig. 2b ). As shown in Fig. 2c , the membrane is free-standing after dehydration. We also confirmed that the membrane was composed of RNA by staining with SYBR Green II ( Fig. 2d,e ). To further characterize our membrane, it has been analysed by energy dispersive X-ray spectrometry and X-ray diffraction, indicating that the membrane was composed of RNA strands and amorphous structure ( Supplementary Figs 4 and 5 ). The micro-scale features of the membrane were observed by both fluorescent and bright-field microscopy, showing a thin folded layer ( Fig. 2e and Supplementary Fig. 6 , respectively). To examine the internal structure and molecular level structure of our RNA membrane, high-magnification images of a scanning electron microscope (SEM) and atomic force microscope (AFM) were also obtained ( Fig. 2f and Supplementary Fig. 7 , respectively). The membrane exhibited micro-scale thickness. As shown in Supplementary Fig. 7 , the membrane has a very smooth surface in nanometre-scale, suggesting compact internal structure of RNA molecules. We also confirmed the native structure of the membrane by liquid-phase AFM imaging. Compared with air AFM images, we could not find any significant difference ( Supplementary Fig. 8 ). In addition, we confirmed that the membrane maintained its original form from repeated dehydration and rehydration ( Supplementary Fig. 9 ). 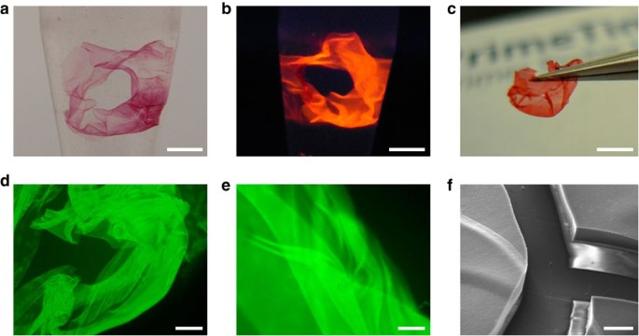Figure 2: Characterization of the self-assembled RNA membrane. Digital camera images of the RNA membrane stained with GelRed (a), under UV light (b) and after dehydration (c). Fluorescent microscopy images of SYBR Green II-stained RNA membrane (dande). SEM image of self-assembled RNA membrane (f). Scale bars, 2 mm ina–c, 50 μm indand 10 μm ine–f. Figure 2: Characterization of the self-assembled RNA membrane. Digital camera images of the RNA membrane stained with GelRed ( a ), under UV light ( b ) and after dehydration ( c ). Fluorescent microscopy images of SYBR Green II-stained RNA membrane ( d and e ). SEM image of self-assembled RNA membrane ( f ). Scale bars, 2 mm in a – c , 50 μm in d and 10 μm in e – f . Full size image Tuning the RNA membrane by partially cRCT We selectively tuned the microstructures by changing the degree of base pairing of the RNA strands. More specifically, by preparing two partially complementary circular DNA for RCT, a process known as partially cRCT (pcRCT), we produced RNA membranes that appeared to have a rough surface and pores ( Fig. 3a ). Interestingly, the membrane was composed of several thin layers ( Fig. 3b ). In addition, a cross-section SEM image of the membrane showed a densely packed internal structure with nanometre-sized RNA grains ( Fig. 3c,d ). To further examine the dependency of the RNA membrane characteristics on the degree of base pairing, we prepared a totally complementary RNA membrane (TCRM) composed of RNA strands that were completely complementary except in the promoter region, with 71 base pairs per repeat unit ( Supplementary Fig. 10a ). We also prepared partially complementary RNA membranes containing 24 base pairs (24-PCRM, Supplementary Fig. 10b ) and 8 base pairs (8-PCRM, Supplementary Fig. 10c ) per repeat unit. The morphologies of the RNA membranes in each case were revealed by SEM ( Fig. 4a–c ) and AFM ( Fig. 4d–f ). Figure 4a,b show the relatively smooth surface of the membrane. 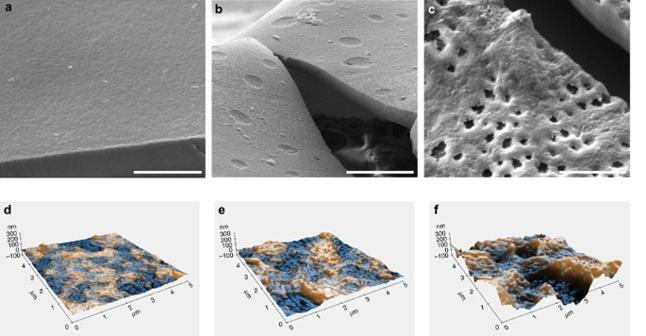Figure 4: Surface properties of totally or partially complementary RNA membranes. SEM images of TCRM, 24-PCRM and 8-PCRM (a–c) and AFM images of TCRM, 24-PCRM and 8-PCRM (d–f) containing 71, 24 and 8 base pairs per repeat unit, respectively. Scale bars, 10 μm ina–c. Interestingly, many craters were observed on the surface of the 24-PCRM ( Fig. 4b ). Moreover, the RNA strands from the eight-base-pair pcRCT formed immature RNA membranes with significant porous structures ( Fig. 4c ). The AFM images of the RNA membranes also suggest that their roughness can be controlled by the degree of base pairing ( Fig. 4d–f and Supplementary Fig. 11a–c ). Young’s modulus of the membranes was also measured by AFM ( Supplementary Fig. 11d ). As we expected, Young’s modulus of 8-PCRM is significantly low in comparison with values of the other two membranes. In addition, we confirmed the thermal behaviour of the membranes with Real-time PCR ( Supplementary Fig. 12 ). Because double-stranded RNA in the membrane will be partially or totally denatured into single strands by heating, intercalated SYBR Green II molecules will be released from the membrane during thermal denaturation process, causing decrease of fluorescent intensity. All three membranes showed different thermal denaturation behaviours, supporting that the character of membrane could be controlled by degree of base pairing. The thickness of the membrane was also dependent on the concentration of the circular DNA. High-magnification SEM images of the RNA membrane with 3 μM of circular DNA revealed that the membrane was approximately 6 μm thick ( Supplementary Fig. 13a ). The thickness of the membranes with 1.5 and 0.3 μM of circular DNA was approximately 5 and 3 μm, respectively ( Supplementary Fig. 13b,c ), suggesting that reducing the concentration of the circular DNAs decreases the thickness of the membrane. However, the AFM images showed that the roughness was not dependent on the concentration of circular DNA ( Supplementary Fig. 13d–f ). 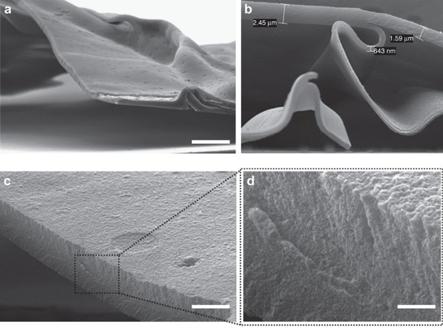According to these results, the roughness, Young’s modulus, thermal behaviour and thickness of the RNA membrane can be rationally controlled by varying the type or concentration of circular DNAs. Figure 3: SEM images of the partially complementary RNA membrane (24-PCRM). Low magnification SEM image for showing free-standing RNA membrane (a) and the thickness of RNA membrane (b). High-magnification cross-section images of RNA membrane (candd). Scale bars, 20 μm, 2 μm and 500 nm ina,candd, respectively. Figure 3: SEM images of the partially complementary RNA membrane (24-PCRM). Low magnification SEM image for showing free-standing RNA membrane ( a ) and the thickness of RNA membrane ( b ). High-magnification cross-section images of RNA membrane ( c and d ). Scale bars, 20 μm, 2 μm and 500 nm in a , c and d , respectively. Full size image Figure 4: Surface properties of totally or partially complementary RNA membranes. SEM images of TCRM, 24-PCRM and 8-PCRM ( a – c ) and AFM images of TCRM, 24-PCRM and 8-PCRM ( d – f ) containing 71, 24 and 8 base pairs per repeat unit, respectively. Scale bars, 10 μm in a – c . Full size image Degradation of RNA membranes in RNase-rich condition After staining the membranes with RNA staining dye (GelRed) ( Supplementary Fig. 14 ), the enzymatic degradation was monitored by measuring the fluorescent intensity of the dyes released in solution ( Fig. 5a ) and observing the deformation of the membranes (inset of Fig. 5a ). Because our membrane was designed to be composed of RNA strands, we carried out the degradation experiments with RNases for 24 h at 37 °C. As a control, RNA membrane was also incubated with DNases and nuclease-free water for 24 h at 37 °C. As expected, the RNA membrane was degraded by RNases, indicating that the membrane was composed of RNA (inset of Fig. 5a ). The membranes incubated with DNases or nuclease-free water seemed to remain intact and maintained their original membrane form (inset of Fig. 5a ). Measuring the fluorescent intensity of the solution confirmed that the membrane was degraded by only RNases. As shown in Fig. 5a , the intensity of the fluorescence increased after 3 h. However, the results did not show any significant increase in fluorescent intensity during incubation in DNase solution and nuclease-free water, suggesting that our membrane was stable and degradable only by its specific nuclease enzyme. Although our RNA membrane was degraded in RNase-rich environment, it could be relatively stable in cell culture condition compared with naked RNA strands. To verify the stability of the membrane in vitro test condition, RNA membranes were incubated in serum (5 or 10%) for 24 h. After incubation, the membranes in 10% serum was separated to several fragments but still was protected from total degradation ( Supplementary Fig. 15a ) and the membranes in 5% serum maintained their original forms for 24 h ( Supplementary Fig. 15b ). In high concentration buffer (10 × TAE buffer, 0.4 M Tris-acetate and 10 mM EDTA), the membrane was also intact after 24 h incubation ( Supplementary Fig. 15c ). 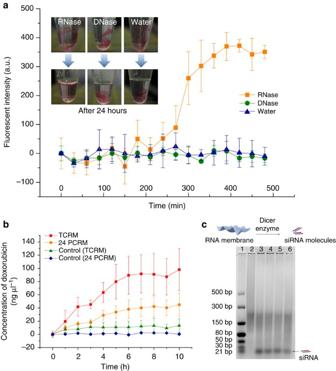Figure 5: Enzymatic degradation of RNA membranes. (a) Degradability of the RNA membrane in RNase solution (orange squares), DNase solution (green circles) and nuclease-free water (blue triangles). The increase of fluorescent intensity in supernatant indicates the degradation of membranes. Digital camera images of stained RNA membranes before reaction (upper images of inset) and after treated with RNase, DNase and nuclease-free water (lower images of inset). (b) Drug release from doxorubicin-loaded TCRM (red squares) and 24-PCRM (orange circles) by RNase. Doxorubicin-loaded TCRM (green triangles) and 24-PCRM (blue diamonds) in nuclease-free water used as controls. (c) Gel electrophoresis result of the generation of siRNA molecules from RNA membrane by Dicer reaction. Lane 1 and 2 indicate double-stranded RNA ladder and RNA membrane without Dicer reaction, respectively. Lanes 3–6 correspond to 12, 24, 36 and 48 h of incubation, respectively. Gel electrophoresis was performed on a 3% agarose gel at 80 V for 2 h with TAE buffer, pH 8.3. a.u., arbitrary unit. Figure 5: Enzymatic degradation of RNA membranes. ( a ) Degradability of the RNA membrane in RNase solution (orange squares), DNase solution (green circles) and nuclease-free water (blue triangles). The increase of fluorescent intensity in supernatant indicates the degradation of membranes. Digital camera images of stained RNA membranes before reaction (upper images of inset) and after treated with RNase, DNase and nuclease-free water (lower images of inset). ( b ) Drug release from doxorubicin-loaded TCRM (red squares) and 24-PCRM (orange circles) by RNase. Doxorubicin-loaded TCRM (green triangles) and 24-PCRM (blue diamonds) in nuclease-free water used as controls. ( c ) Gel electrophoresis result of the generation of siRNA molecules from RNA membrane by Dicer reaction. Lane 1 and 2 indicate double-stranded RNA ladder and RNA membrane without Dicer reaction, respectively. Lanes 3–6 correspond to 12, 24, 36 and 48 h of incubation, respectively. Gel electrophoresis was performed on a 3% agarose gel at 80 V for 2 h with TAE buffer, pH 8.3. a.u., arbitrary unit. Full size image Inspired by the advantages of RNA membranes, we explored the potential of our RNA membrane for use in an enzyme-responsive drug-release system ( Fig. 5b ). We loaded chemotherapy drug, doxorubicin (DOX), to our RNA membrane with high-loading efficiency (up to 98%) through intercalation process ( Supplementary Fig. 14 ). Both two RNA membranes, TCRM and 24-PCRM were examined. Figure 5b shows the enzymatically responsive release profiles of DOX from these two membranes. By introducing RNase to the membranes, relatively smooth release curves were observed. As expected, the release of DOX was dependent on the type of membrane used. These release differences may be attributed to membrane characteristics such as roughness and thickness. No significant increases were detected from the TCRM and 24-PCRM in water, confirming the drug release by enzymatic reaction. To further explore the usage of RNA membrane, we examined the potential for efficient siRNA release. Our membrane consists of RNA strands and can be processed by Dicer, endoribonuclease that cleaves double-stranded RNA into 21–25 bp long potential siRNAs. To confirm the generation of siRNA molecules, RNA membranes were incubated with recombinant Dicer and then the results were analysed by gel electrophoresis. As shown in Fig. 5c , generation of siRNA from the membranes was successfully achieved in the presence of Dicer (lane 3–6 of Fig. 5c ). We have demonstrated the fabrication of an RNA-based membrane that can be rationally manipulated. We also suggested a general approach for generating macroscopic RNA materials that cannot be achieved with currently available methods. To the best of our knowledge, this is the first report describing an enzymatically produced RNA membrane that is large enough to be observed with the naked eye. In addition, this macroscopic RNA membrane could be produced at a much lower cost than using commercially synthesized RNA molecules. These enzymatically produced RNA strands can provide much richer options for constructing self-assembling RNA structures. Two fundamental mechanisms contribute to the generation of self-assembled two-dimensional RNA structures. One mechanism is through cRCT, which produces two complementary RNA strands through the formation of a thin ring-like structure as a seeding material. The other mechanism is through the self-assembly of RNA strands by evaporation. The EISA process is mainly achieved by the concentration and hybridization of RNA strands. Therefore, the degree of RNA base pairing has an important role in determining the characteristics of RNA membranes. Characterization of the RNA membranes suggests that their roughness, Young’s modulus and thermal stability can be controlled by the degree of base pairing. The thickness of the membranes was also determined by varying the concentration of circular DNA, which was related to the concentration of RNA strands. The adaptability of RNA membranes and the nature of RNA itself bolster its potential for various applications, including the release of chemicals and siRNA. For example, RNA membranes have been used for chemical molecule release, suggesting the potential as a patch in industrial application. In addition, engineered nanoscale RNA membranes could be effective siRNA delivery carrier. In this study, we successfully introduced an approach for RNA-assembly on a macro-scale. Although further improvements for real-world application are needed, our RNA membrane presents a new route for RNA technology. Circularization of long linear DNA DNA oligonucleotides were purchased from Integrated DNA Technologies (IDT). To synthesize 1 μM of circular DNA, phosphorylated long linear DNA (final concentration of 1 μM) and T7 promoter DNA (final concentration of 1 μM) were mixed in nuclease-free water. For denaturation and annealing, the mixed solution was heated at 95 °C for 2 min and slowly cooled to 25 °C for 1 h using a PCR thermal cycler (Bio-Rad). To ligate the nick in the circularized DNA, the solution was incubated overnight with 0.03 U μl −1 of T4 ligase (3 U μl −1 , Promega) and ligase buffer (300 mM Tris-HCl (pH 7.8), 100 mM MgCl 2 , 100 mM dithiothreitol and 10 mM adenosine triphosphate) at room temperature. Next, 1 μM of circular DNA was concentrated to 10% of its original volume for further processes using a concentrator or centrifugal filter (YM-3, Millipore). Self-assembly of RNA membranes using cRCT and EISA To prepare the reaction solution for cRCT, circular DNA (final concentration of 3 μM) and complementary circular DNA (final concentration of 3 μM) were mixed with 3.75 mM of ribonucleotide solution mix (New England Biolabs), reaction buffer (8 mM Tris-HCl, 0.4 mM spermidine, 1.2 mM MgCl 2 and 2 mM dithiothreitol) and 5 U μl −1 of T7 RNA polymerase (50 U μl −1 , New England Biolabs). For the cRCT process, the reaction solution was incubated for 20 h at 37 °C. After the cRCT process, the cap of the tube was opened to initiate the EISA process. The tube was incubated overnight at 37 °C. Relative humidity should be considered for effective EISA process ( Supplementary Fig. 16 ). In this study, we fabricated the membrane at 25% relative humidity. Degradation of RNA membranes For staining, the RNA membrane was prepared with 2 μl of RNA staining dye (GelRed or SYBR Green II) in nuclease-free water (final volume of 100 μl) and incubated overnight at room temperature. To rinse the membrane and remove the free GelRed molecules, the existing solution was exchanged three times with fresh nuclease-free water. For the degradation experiment, stained RNA membranes were prepared with RNases (0.1 U μl −1 of RNase III and 0.1 U μl −1 of RNase I, Epicentre) or DNases (1 U μl −1 of Exonuclease III and 1 U μl −1 of Exonuclease I, Epicentre) in nuclease-free water (final volume of 100 μl). The membranes were incubated for 24 h at 37 °C. To measure the degrees of degradation of the membranes, the solutions were analysed at 30-min intervals by a micro-plate reader (BioTek, Model: Synergy HT). Drug release from RNA membranes To load DOX (5 μg μl −1 , Sigma Aldrich) into the membrane, 2 μl of DOX was added to the membrane with 98 μl of nuclease-free water, and the membrane was incubated overnight at 4 °C. After incubation, free DOX was removed and the membrane was washed with nuclease-free water. To release DOX from the membrane, DOX-loaded RNA membrane was prepared with RNases (0.025 U μl −1 of RNase III and 0.025 U μl −1 of RNase I, Epicentre) in nuclease-free water (final volume of 100 μl) at 37 °C. The fluorescent intensity was measured to determine the degree of DOX release by a micro-plate reader (BioTek, Model: Synergy HT). Treatment of RNA membrane with Dicer for siRNA release To cleave the membrane to small fragments, the membrane was sonicated for 10 min using bath sonicator (SD Ultra Sonic Cleaner) with 28 kHz ultrasonic frequency. The RNA membranes were then incubated with 1 unit of recombinant Dicer (Genlantis) and reaction solution (1 mM adenosine triphosphate, 2.5 mM MgCl 2 , 40% Dicer reaction buffer) in nuclease-free water (final volume of 10 μl) for generating 21-bp siRNA molecules. To optimize the reaction time for siRNA generation, the membrane samples were incubated with different reaction times from 12 to 48 h at 37 °C. After incubation, 2 μl of Dicer Stop Solution (Genlantis) was added to deactivate Dicer. Generated siRNA molecules were then confirmed by gel electrophoresis with 3% agarose gel. How to cite this article: Han, D. et al. Self-assembly of free-standing RNA membranes. Nat. Commun. 5:4367 doi: 10.1038/ncomms5367 (2014).